Slow-light-enhanced gain in active photonic crystal waveguides Passive photonic crystals have been shown to exhibit a multitude of interesting phenomena, including slow-light propagation in line-defect waveguides. It was suggested that by incorporating an active material in the waveguide, slow light could be used to enhance the effective gain of the material, which would have interesting application prospects, for example enabling ultra-compact optical amplifiers for integration in photonic chips. Here we experimentally investigate the gain of a photonic crystal membrane structure with embedded quantum wells. We find that by solely changing the photonic crystal structural parameters, the maximum value of the gain coefficient can be increased compared with a ridge waveguide structure and at the same time the spectral position of the peak gain be controlled. The experimental results are in qualitative agreement with theory and show that gain values similar to those realized in state-of-the-art semiconductor optical amplifiers should be attainable in compact photonic integrated amplifiers. Slow light is a fascinating physical effect, raising fundamental questions related to our understanding of light–matter interactions as well as offering new possibilities for photonic devices. From the first demonstrations of slow-light propagation in ultra-cold atomic gasses [1] , solid-state Ruby [2] and photonic crystal (PhC) structures [3] , focus has shifted to applications, with slow light offering the ability to enhance and control light–matter interactions. The demonstration of tuneable delay lines [4] , [5] , [6] , enhanced nonlinearities [7] , [8] and spontaneous emission [9] , enlarged spectral sensitivity [10] and increased phase shifts illustrate the possibilities enabled by slow-light propagation, with microwave photonics emerging as one of the promising applications [11] . Stimulated emission of radiation leads to the amplification of a propagating electromagnetic wave, forming the basis for optical amplifiers and lasers. The strength of the process is quantified by the gain coefficient per unit length, and is usually considered to be governed by the material properties. Dowling et al . [12] suggested that the slow down of light near the edge of a one-dimensional photonic bandgap structure could be used to enhance the gain coefficient. The slow propagation of the Bloch mode near the band edge, which may be visualized as multiple back-and-forth scattering of the light beam, thus lengthens the local dwell time in the medium and increases the spatial but not the temporal gain coefficient [13] . Despite obvious applications in optical amplifiers [14] , [15] and lasers [16] , there is no conclusive experimental demonstration in a waveguide structure. For dye-doped three-dimensional artificial opals, enhancement of gain in certain crystallographic directions and its relation to the directional density of optical states was demonstrated [17] , and in ref. 18 enhancement effects in multimode InP waveguides related to a ministop band were indicated. Spontaneous emission enhancement was observed in PhC wires [19] and dielectric multilayers with oxygen vacancies as light emitters [20] , and may be used to increase the spontaneous emission factor of a waveguide [9] . Early measurements on lasers employing PhC waveguides [21] , [22] and coupled resonator structures [23] show that the lasing characteristics are improved using slow-light effects. However, as both the cavity quality factor and the spatial gain coefficient may be affected by slow-light propagation, laser measurements cannot easily distinguish between the two effects. Thus, measurements on open structures are required. In this study we experimentally demonstrate that the gain of an active waveguide can indeed be enhanced using slow-light effects in PhCs, enabling compact linear and nonlinear devices suitable for photonic integration, as well as providing opportunities for spectral and spatial control of the gain. The effect was theoretically predicted but not yet experimentally demonstrated. The maximum achievable gain is limited by amplified spontaneous emission, as well as multiple-scattering and localization due to disorder. Theory of slow-light-enhanced gain Before describing our experimental results, we briefly summarize the theoretical status. An extensive analysis for a periodic PhC lattice shows that the gain scales with the density of optical states [16] . For a one-dimensional defect waveguide, based on qualitative considerations of the effective path length, Dowling et al . [12] suggested a linear scaling of gain with group index. By expansion into Bloch waves, we derived the following approximate expression for the modal gain coefficient (see Supplementary Methods ) with g mat being the material gain, g 0 the bare material gain in absence of a PhC waveguide, n g the group index, n b the background refractive index of the active material and Γ a generalized confinement factor describing the field overlap with the active material. The importance of the latter was demonstrated experimentally in absorption-type measurements [24] . Equation (1) agrees with the result of a perturbative analysis [25] . The predicted scaling of the modal gain (or absorption) with group index has, despite its intuitive appeal, been the subject of some controversy, and it was shown that one needs to distinguish between slow light originating from structural perturbations, for example a PhC waveguide, and material dispersion, such as electromagnetically induced transparency [26] . For the latter, equation (1) does not hold, as also demonstrated experimentally [27] . Moreover, for translationally invariant systems, such as a fibre, the gain enhancement due to slow light induced by mode dispersion is exactly cancelled by the resulting transversal expansion of the mode [26] . To confirm equation (1) and quantify the impact of slow light on the modal gain, we carried out extensive calculations of gain spectra in different structures, see Fig. 1 . As the mode frequency ( Fig. 1a ) approaches the band edge, the group index ( Fig. 1b ) of the PhC waveguide strongly increases, leading to a significant increase of the modal gain coefficient of the corresponding active PhC waveguide ( Fig. 1c , a =380 nm). Gain spectra for two other PhC lattice constants and the same electronic density of states and carrier distributions are also shown. The gain spectra may be compared with that of a rectangular waveguide (nanowire) embedded in air, which is proportional to the material gain spectrum and has a confinement factor similar to the PhC structures (~40%, see Supplementary Fig. 1 for additional detail). In Fig. 1d , the gain enhancement factor is shown as a function of the group index. The enhancement factor is defined as the modal net gain of the PhC waveguide divided by the modal gain of the nanowire waveguide, (Γ g 0 n g / n b − α )/(Γ ref g 0 ), where Γ ref is the confinement factor of the reference waveguide and α is the loss of the PhC waveguide (see Supplementary Methods ). Notice that this provides a conservative estimate of the gain enhancement, as losses in the reference waveguide are neglected. The dashed line in Fig. 1d indicates the linear scaling with group index that is obtained when the impact of structure disorder is neglected. For the regime of large group index (approximated by n g >40, shaded grey), disorder limits the maximum gain enhancement factor that can be reached. Close to the transparency wavelength around 1,500 nm, where the net gain is zero, additional waveguide loss in the PhC waveguide slightly shifts the transparency wavelength for the net gain. As the group index at the transparency point is larger for the structures with larger lattice constant, the gain enhancement in this spectral region is smaller for those structures. 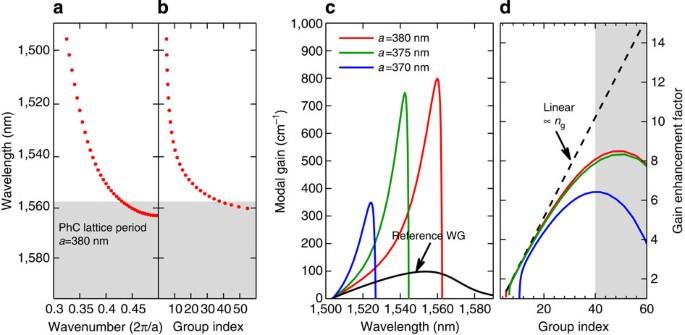Figure 1: Comparison of calculated modal gain in standard and slow-light-enhanced waveguides. (a) Photonic band diagram and (b) corresponding group index of the passive three-dimensional PhC waveguide for TE-like modes. (Triangular lattice of air holes witha=380 nm,r=0.26a,h=340 nm,, ten layers of 10 nm QWs placed in the middle of membrane). In the grey area, the gain is impacted by slow-light-enhanced scattering loss due to disorder. (c) Modal gain spectra (including disorder-induced losses) of fundamental transverse electric (TE)-like modes for three 10 QW PhC waveguides with lattice periods of 380, 375 and 370 nm, as well as for a reference rectangular waveguide with 10 QWs (width 660 nm, height 340 nm,, group index 3.8, and confinement factor of 40%). (d) Gain enhancement factor as function of group index. Dashed line indicates the linear scaling with group index when the impact of structure disorder is neglected. Figure 1: Comparison of calculated modal gain in standard and slow-light-enhanced waveguides. ( a ) Photonic band diagram and ( b ) corresponding group index of the passive three-dimensional PhC waveguide for TE-like modes. (Triangular lattice of air holes with a =380 nm, r =0.26 a , h =340 nm, , ten layers of 10 nm QWs placed in the middle of membrane). In the grey area, the gain is impacted by slow-light-enhanced scattering loss due to disorder. ( c ) Modal gain spectra (including disorder-induced losses) of fundamental transverse electric (TE)-like modes for three 10 QW PhC waveguides with lattice periods of 380, 375 and 370 nm, as well as for a reference rectangular waveguide with 10 QWs (width 660 nm, height 340 nm, , group index 3.8, and confinement factor of 40%). ( d ) Gain enhancement factor as function of group index. Dashed line indicates the linear scaling with group index when the impact of structure disorder is neglected. Full size image It is well known that as the band edge is approached, scattering losses are enhanced due to slow-light propagation [28] , [29] , [30] , [31] . This loss enhancement was included phenomenologically using a third-order polynomial dependency on n g . We note that, typically, a second-order polynomial is assumed where the squared term accounts for the backscattering losses and the linear term accounts for out-of-plane losses. However, as noted in refs 28 , 29 , 30 , 31 , for passive photonic crystal waveguides (PCW) this is a crude model, as it does not account for the mode shape being dependent on n g . The assumed third-order dependency may partially account for this mode-shape dependency. Throughout the remainder of this work, we shall refer to the modal gain minus waveguide losses as the net gain, g . These results thus predict that the net gain can be enhanced and controlled via the photonic environment rather than the usual approach of modifying the epitaxial structure. Measurement of slow-light-controlled gain spectra PhC waveguides with one missing air hole (W1 type) are fabricated in a 340-nm-thick air-embedded InGaAsP membrane with a triangular-lattice pattern of air holes (see Methods). The waveguide is terminated by tapers [32] to suppress residual reflections and improve coupling. Similar passive structures have been used for investigating slow-light propagation [3] , [4] and nonlinearities [7] , [8] , but in our case an active material is incorporated inside the membrane and the structures are designed such that the slow-light regime spectrally overlaps with the region where positive net material gain can be achieved by optical pumping. A schematic of the setup as well as scanning electron microscopy pictures of fabricated samples are shown in Fig. 2 . Figure 3 shows measured spontaneous emission spectra for three 1-mm-long waveguides with different PhC lattice parameters, corresponding to a progressive wavelength shift of the slow-light region by 20 nm. 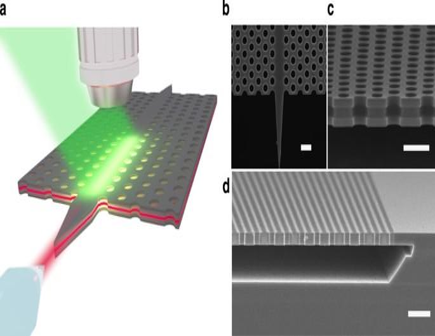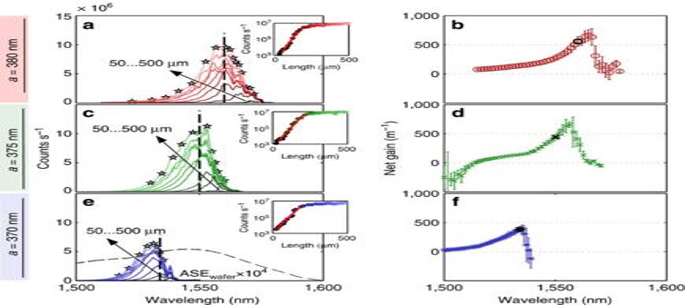Figure 3: Slow-light-enhanced spontaneous emission and gain spectra. Amplified spontaneous emission spectra (a,c,e) for varying pump stripe length (for clarity, only spectra for every 50 μm are shown) and derived net gain versus wavelength (b,d,f) for three 10 QW PhC waveguides with lattice constants of 380 nm (a,b), 375 nm (c,d) and 370 nm (e,f). The insets show the intensity versus stripe length and the corresponding fits for the wavelengths indicated by vertical dashed lines. The extracted gain value is indicated by a black marker in the gain spectra (b,d,f). The star markers (a,c,e) indicate spectral features in the spectra that are used for extracting an optical path length (cf.Fig. 4). Figure 2: Measurement set-up and structures investigated. (a) Schematic of the active membrane exposed to a focused pump beam (green) and the fibre collecting light from the taper. Scanning electron microscopy images showing (b) the taper (scale bar, 500 nm (white)), (c) the active material in the centre of the membrane (scale bar, 500 nm) and (d) the PhC membrane (scale bar, 1 μm). Figure 2: Measurement set-up and structures investigated. ( a ) Schematic of the active membrane exposed to a focused pump beam (green) and the fibre collecting light from the taper. Scanning electron microscopy images showing ( b ) the taper (scale bar, 500 nm (white)), ( c ) the active material in the centre of the membrane (scale bar, 500 nm) and ( d ) the PhC membrane (scale bar, 1 μm). Full size image Figure 3: Slow-light-enhanced spontaneous emission and gain spectra. Amplified spontaneous emission spectra ( a , c , e ) for varying pump stripe length (for clarity, only spectra for every 50 μm are shown) and derived net gain versus wavelength ( b , d , f ) for three 10 QW PhC waveguides with lattice constants of 380 nm ( a , b ), 375 nm ( c , d ) and 370 nm ( e , f ). The insets show the intensity versus stripe length and the corresponding fits for the wavelengths indicated by vertical dashed lines. The extracted gain value is indicated by a black marker in the gain spectra ( b , d , f ). The star markers ( a , c , e ) indicate spectral features in the spectra that are used for extracting an optical path length ( cf . Fig. 4 ). Full size image The devices have identical ten quantum-well (QW) epitaxial structures and the measurements thus clearly show that the emission spectrum can be controlled via the PhC lattice parameters. The different spectra shown for each of the samples correspond to different excitation stripe lengths, defined by blocking part of the pump light in close vicinity to the sample. If the modal gain exceeds the total losses, the spontaneous emission is amplified along the waveguide. To measure the net gain, including propagation losses due to non-resonant residual absorption as well as disorder-induced scattering, we use a standard method originally introduced in the seminal work of Shaklee et al . [33] The output intensity may be written as where l is the excitation stripe length and A is proportional to the local rate of spontaneous emission. To measure the gain, we fitted the data using the normalized function I ( l )/ I ( L ), which is independent of A , where L is a reference length given by the longest length included in the fit. Inserts in Fig. 3 show example variations of intensity with stripe length, with the intensity increasing by more than three orders of magnitude, and the corresponding fits. For long stripe lengths, the intensity saturates, the origin of which is discussed later, and this part is omitted in the fit (see Methods for details). Figure 3 shows the extracted gain spectra for the three waveguides under similar pumping conditions. The spectra are seen to shift in good qualitative agreement with the simulations shown in Fig. 1c . Our measurement scheme avoids the problem of Fabry–Perot resonances induced by facet reflections, as the far-side facet is preceded by unpumped material with strong absorption. The caveat is that due to the absence of a well-defined cavity, we do not have access to independent measurements of the absolute group index variation of the structures. To confirm that our waveguides do display the generally accepted variation of group index with wavelength [28] , [29] , [31] , we present in Fig. 4 the measured emission spectrum of a structure with a =380 nm and r / a =0.25 (same as the waveguide plotted in red in Fig. 3 ) but implementing a 10-μm-long PhC cavity by terminating the waveguide at both ends by holes. A tenfold light slow down is observed close to the band edge of this device. The slight shift in band edge position, compared with the samples in Fig. 3 , is related to the lower relative permittivity of this waveguide, which contains one layer of quantum dots instead of ten QWs. To get information on the location of the band edge for the exact same samples as investigated in Fig. 3 , we analyse the fringe spacing, δλ , in the spectra, most clearly noticed for the sample with a =380 nm close to the band edge. We attribute these fringes to imperfections in the lattice that cause reflections. We may calculate the variation of the optical path length as n g L = λ 2 /(2 δλ ). To estimate the absolute value of the group index, we compare with the measured group index of the reference QD sample in Fig. 4 . Assuming the wavelength dependence of the group index to be the same for the reference sample and the samples used in the gain spectra measurements, which is reasonable considering that they are nearly identical except for absolute shifts of the band edge, we calibrate the group indices for the shortest wavelengths, n g ( λ < ), to be 6.5, 9 and 11, for the three structures. Using this, we may estimate the group indices as n g ( λ ) L /[ n g ( λ < ) L ]· n g ( λ < ), giving a maximum n g of 40–50, see Fig. 4a , corresponding to slow-down factors of 11–14. The position of the band edge extracted from these measurements correlate well with the position at which the measured gain spectra attain their maxima, cf . Fig. 3 , thus confirming that the gain enhancement is a slow-light effect. Moreover, the magnitudes of the calculated group indices near the band gap are in good agreement with the measured group index of the terminated waveguide structure in Fig. 4 (bottom). Comparing the estimated slow-down factor with the calculated gain enhancement in Fig. 1d , we notice that the latter is slightly smaller, as is expected from the slow-down enhancement of the propagation losses. We have also performed transmission measurements (see Supplementary Fig. 4 ) confirming that the maximum transmission varies according to the PhC band edge. 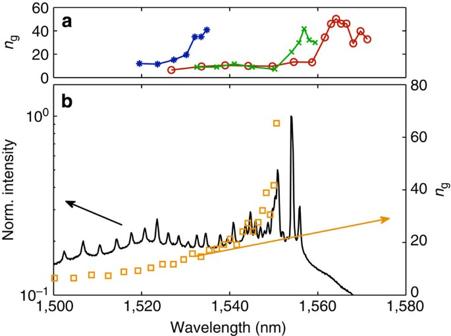Figure 4: Measured group index and position of band-gap edge. (a) Group indices extracted from emission spectra shown inFig. 3for the lattice constants 380 nm (red circles), 375 nm (green crosses) and 370 nm (blue asterisks). (b) Measured amplified spontaneous emission spectrum and group index for a 10-μm-long cavity in a PhC slab witha=380 nm andr/a=0.25. Figure 4: Measured group index and position of band-gap edge. ( a ) Group indices extracted from emission spectra shown in Fig. 3 for the lattice constants 380 nm (red circles), 375 nm (green crosses) and 370 nm (blue asterisks). ( b ) Measured amplified spontaneous emission spectrum and group index for a 10-μm-long cavity in a PhC slab with a =380 nm and r / a =0.25. Full size image Saturation effects As mentioned, the output intensity is observed to saturate beyond a certain length, L max , (see Methods). 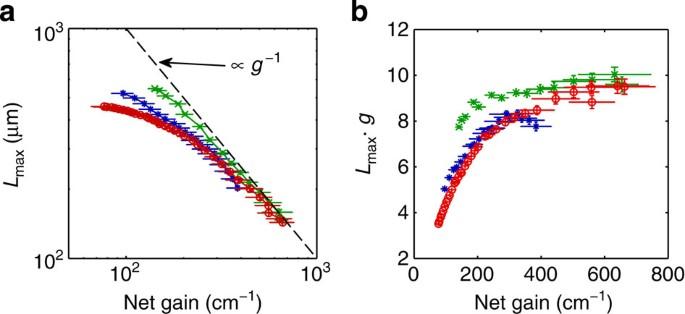Figure 5: Saturation effects. (a) Extracted maximum stripe length,Lmaxas a function of extracted net gain. The dashed line is a guide to the eye being inversely proportional to the net gain. (b) Extracted gain-length product as a function of net gain. Colors indicate different PhC structures, seeFig. 3. Figure 5a shows the variation of L max as a function of measured net gain. The maximum stripe length is observed to decrease with increasing gain, and for large gain values L max is seen to scale inversely with gain. By plotting the gain-length product, gL max , versus net gain ( Fig. 5b ), we find that gL max saturates at a value of 8–9, corresponding to a maximum gain of 35–39 dB. This is in good qualitative agreement with findings for bulk amplifiers [34] , where a maximum gain of about 34 dB, limited by amplified spontaneous emission, was found. We also notice that for a given structure, the product gL max decreases for small gain values. This is consistent with the attribution of gain saturation to amplified spontaneous emission (ASE). The depletion of the carrier density thus lowers the Fermi levels for conduction and valence bands, and the gain therefore decreases more readily at shorter wavelengths than at longer wavelengths, where the occupation probabilities are close to 1. We take these observations as strong indications that the saturation of the intensity with stripe length is due to carrier depletion and subsequent gain reduction due to amplified spontaneous emission. Notice that the carrier density may also be reduced due to lasing in random cavities formed due to unintentional structural disorder, as discussed later. The prospect of slow-light amplifiers is thus not to increase the absolute gain, but rather to provide high gain in a short device, as required for photonic integration. Figure 5: Saturation effects. ( a ) Extracted maximum stripe length, L max as a function of extracted net gain. The dashed line is a guide to the eye being inversely proportional to the net gain. ( b ) Extracted gain-length product as a function of net gain. Colors indicate different PhC structures, see Fig. 3 . Full size image In the presence of disorder, multiple scattering events may dominate the propagation of light for long stripe lengths, thus invalidating the Beer–Lambert expression on which equation (2) is based (see ref. 31 ). Although, in our case, amplified spontaneous emission appears to be the governing cause of saturation, the role of disorder could be experimentally investigated by introducing deliberate, random disorder in the PhC structures. With present technology, passive PhC waveguides exhibit a propagation loss of ~2 dB mm −1 in the conventional ‘fast-light’ region, while propagation losses strongly depend on n g in the slow-light regime [28] . Even though the propagation loss therefore is much higher than for well-designed ridge waveguides, a positive net gain coefficient up to ~700 cm −1 is measured ( Fig. 3 ). Gain spectra of electrically contacted standard ridge waveguides, with five QWs of the same composition and thickness as employed here were measured to have a maximum gain of 10 cm −1 per QW, thus revealing a gain enhancement of roughly 700/(10 × 10)=7. Here, a factor ~2 is expected from the tighter confinement of the waveguide (see Supplementary Methods ) and the remaining factor ~3.5 can thus be ascribed to slow-light enhancement. From Fig. 4 , a slow-light enhancement factor of ~8 at the measured group index of ~50 is expected, when comparing with a reference waveguide of nearly the same confinement factor as the PhC waveguide. The lower experimental enhancement factor is most likely to be due to additional heating and higher carrier loss due to surface recombination in the PhC waveguide structures as well as multiple-scattering effects due to fabrication disorder. However, recent work has demonstrated the feasibility of realizing a buried heterostructure and electrical pumping [35] , which will strongly reduce these limitations. Furthermore, dispersion engineering [4] may be applied to optimize the group index variation relative to the gain peak. From the gain spectra in Fig. 3 , one notices that the transparency point (where the net gain is zero) appears blue shifted for the smallest PhC lattice periodicity. This indicates that the resulting carrier density is higher for that structure despite the near-identical pumping conditions and is likely to be due to suppression of spontaneous emission at longer wavelengths caused by the photonic bandgap. This suggests a way of increasing the quantum injection efficiency into the desired levels without changing the electronic level structure and would be very interesting from a pump efficiency point of view. So far, such tailoring was accomplished by exploiting quantum confinement effects in low-dimensional semiconductors. Further investigations with improved measurement accuracy and implementation of electrical pumping are, however, required to conclude on this, and three-dimensional PhC structures are desirable for exercising complete suppression of undesired recombination channels. Similar to conventional semiconductor optical amplifiers, the gain of a PhC amplifier will be limited by carrier depletion caused by the injected signal or by amplified spontaneous emission. Slow-light propagation may cause additional effects. As already mentioned, random scattering due to fabrication-induced disorder reduces the maximum attainable group index and increases the loss. As the band edge is approached, local cavities may even form, leading to random lasing [36] . Even in the absence of disorder, distributed feedback (band edge) lasing [22] may set in close to the Brillouin zone edge and these lasing effects will lead to further carrier depletion, thus limiting the maximum gain. It was recently predicted that the slow down of the light itself will be limited by the presence of gain, due to broadening of the optical density of states [37] . This effect, not yet experimentally observed, may also be contributing to the gain saturation that we observe experimentally, but we cannot presently separate that from the effect of gain depletion due to amplified spontaneous emission. In conclusion, we have demonstrated that the gain of a waveguide can be enhanced and spectrally controlled by exploiting slow-light propagation. This is promising for the realization of compact integrated PhC amplifiers, which are essential, presently missing, components for integrated photonic chips. The use of slow light may also reduce the power consumption of amplifiers, as less active material needs to be inverted to achieve a given gain. Furthermore, the control of the gain profile via the photonic structure, rather than the electronic, epitaxial structure, provides new design freedom, for example, allowing varying the gain coefficient along the waveguide, which may be exploited for ultrafast low-power signal processing applications. The present work also demonstrates a platform for fundamental studies of propagation and random scattering effects in structures under the combined effect of slow light and net gain, which are topics that have proved very rich, even for passive structures. Device fabrication The wafers were grown by metal-organic vapour phase epitaxy on InP substrates. The membrane is InGaAsP ( λ g =1.15 μm) with a total thickness of 340 nm containing one or ten strain-compensated QWs (6 nm In 0.75 Ga 0.25 As 0.86 P 0.14 well, 7.2 nm In 0.49 Ga 0.51 As 0.86 P 0.14 barrier) in the centre. Sacrificial layers underneath were formed by a stack of 100 nm InP, 100 nm InAlAs and 800 nm InP with a total thickness of 1 μm. A 200-nm layer of SiN x was deposited by plasma-enhanced chemical vapor deposition (PECVD) followed by a 500-nm-thick layer of a positive e-beam resist (zep520A). The patterning was done using e-beam writing by a JEOL-JBX9300FS. The pattern was transferred to the SiN x by CHF3/O2 reactive ion etch and further transferred to the semiconductor by cyclic CH 4 /H 2 —O 2 reactive ion etch after resist removal. Beneath the active slab, there is a 1 μm-thick sacrificial layer, which is etched away using 1HCl:2H 2 O selective wet-etching to obtain an air-slab structure. Device characterization The devices are optically excited along a stripe by focusing pump laser light onto the waveguide using a cylindrical lens. To avoid effects of heating, the samples are pumped with pulses from a mode-locked Ti:Sapphire laser (wavelength 800 nm, duration ~1 ps, repetition rate 270 kHz) with an average power of 6 mW (corresponding to 40 W cm −2 average power or a pulse fluence of ~1.5 pJ μm −2 ). The stripe width was ~15 μm. The waveguide output is coupled to a lensed fibre using a PhC waveguide taper. A series of spontaneous emission spectra from well-defined excitation stripe lengths are acquired using a cooled InGaAs array detector on a spectrograph. The excitation stripe lengths are measured from calibrated camera microscope images of the spontaneously emitted near infrared light scattered out from the top of the waveguide. Gain extraction and error bar estimation The gain spectrum was extracted by fitting to equation (2) using the maximum likelihood method. Shot noise was found to be negligible and the noise rather resulted from fluctuations due to waveguide–fibre coupling. Accordingly, as the statistical error is proportional to the mean output signal, we assume a log-normal (rather than a normal) distribution corresponding to the logarithm of the output signal being normally distributed. The fits thus minimize the sum of squared residuals for the logarithm of the measured ASE. The error bars shown are the calculated 95% confidence intervals. It might be expected that the uncertainty should be at a minimum where the ASE spectrum peaks, as here the output signal shows the largest variation with stripe length. However, the signal is observed to saturate at a shorter stripe length for higher gain, limiting the useful fitting range where the exponential dependence in equation (2), which neglects saturation, holds true. Examples of fits with indication of the fitting range employed are shown in the insets of Fig. 3 . To systematically determine the fitting range, we carried out fits for all wavelengths versus maximum pump lengths and used the set of wavelengths and fitting ranges resulting in an R 2 value (coefficient of determination), closest to 1. R 2 is a standard measure for the goodness of a fit and was evaluated as R 2 =1− S err /S tot , where S err = ∑ i [ln ( y i )−ln ( I i )] 2 and S tot = ∑ i [ln ( y i )− <ln ( y )>] 2 and y i ( I i ) is the measured ASE with pump stripe length z i . How to cite this article: Ek, S. et al. Slow-light-enhanced gain in active photonic crystal waveguides. Nat. Commun. 5:5039 doi: 10.1038/ncomms6039 (2014).